Suppression of electron–vibron coupling in graphene nanoribbons contacted via a single atom Graphene nanostructures, where quantum confinement opens an energy gap in the band structure, hold promise for future electronic devices. To realize the full potential of these materials, atomic-scale control over the contacts to graphene and the graphene nanostructure forming the active part of the device is required. The contacts should have a high transmission and yet not modify the electronic properties of the active region significantly to maintain the potentially exciting physics offered by the nanoscale honeycomb lattice. Here we show how contacting an atomically well-defined graphene nanoribbon to a metallic lead by a chemical bond via only one atom significantly influences the charge transport through the graphene nanoribbon but does not affect its electronic structure. Specifically, we find that creating well-defined contacts can suppress inelastic transport channels. The atomic-scale details of the contacts in molecular electronics are of crucial importance for the electrical characteristics of the device [1] , [2] , [3] . The contacts are typically realized through specific chemistries by using terminal functional groups, for example, thiols for bonding to gold [4] , [5] . However, these approaches are not necessarily ideal in terms of electrical transparency, mechanical stability and atomic level control over the bonding geometry [5] , [6] , [7] . Atomic-scale control will also be required in contacting graphene nanostructures as their size is scaled down to open a sufficient energy gap between the valence and the conduction bands through quantum confinement for device operation at room temperature [8] , [9] , [10] , [11] , [12] , [13] . It is also critical for realizing novel graphene devices based on theoretically motivated concepts such as valleytronics [14] , [15] . Surprisingly, although graphene nanoribbons (GNRs) have been proposed to be used as molecular scale interconnects and components in graphene-based nanoelectronics, making contacts via metal-carbon bonds has not been examined experimentally. Here, we contact an atomically well-defined GNR [13] , [16] , [17] to the gold substrate by a chemical bond via only one atom. This well-defined contact is formed by removing an individual hydrogen atom from the end of a GNR. We use combined atomically resolved atomic force microscopy (AFM) and scanning tunnelling microscopy (STM) to show that this bond formation strongly suppresses the electron–vibron (e–v) coupling, but does not affect the bulk electronic structure of the GNR. Geometric and electronic structure of the GNRs We have carried out combined low-temperature STM/AFM experiments on atomically well-defined GNRs grown through the on-surface polymerization of 10-10′-dibromo-9,9′-bianthryl followed by thermal cyclodehydrogenation on Au(111) single crystals ( Fig. 1a , see Cai et al. [13] ; Ruffieux et al. [16] ; Koch et al. [17] and Methods for details). A typical overview STM scan is shown in Fig. 1b . Although many of the ribbons are attached to other ribbons or to gold step edges, we also observe individual, free ribbons ( Fig. 1c ). Such free ribbons are mobile, that is, imaging them with current set-points above ~10 pA resulted in lateral motion along the long axis of the GNR. This indicates that defect-free GNRs are only weakly coupled to the substrate, in line with previous experiments on π-conjugated molecules on Au(111) [18] . Atomically resolved constant-height AFM images, acquired with a CO-terminated tip, of the central part and the end of a ribbon are shown in Fig. 1d , respectively. The GNRs have the expected structure based on the synthesis procedure: a series of alternating rows of 3 and 2 fused benzene rings along its long axis and termination in an anthracene moiety. We do not observe any reconstruction of the edges. Hence, the edges and ends correspond to armchair and zigzag termination, respectively. Similar images of an entire ribbon show that the synthesis method typically yields defect-free GNRs. However, defects are sometimes observed. An example is displayed in Fig. 1f , which shows an atomically resolved image of a 22-mer GNR. This ribbon has one missing benzene ring (indicated by the red arrow) that is clearly visible in the AFM ( Fig. 1f ). However, this major modification of the geometric structure is difficult to identify in the corresponding STM image ( Fig. 1g ). This underlines the importance of acquiring simultaneous STM and AFM data. 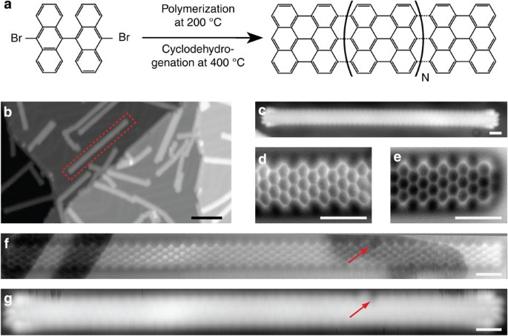Figure 1: Chemical structure of atomically precise graphene nanoribbons. (a) Bottom-up synthesis of an armchair GNR results in zigzag terminated ends. (b) STM overview image showing a free GNR (V=50 mV,I=5 pA). (c) Free GNR imaged with a CO-terminated tip (V=10 mV,I=5 pA). (d,e) Constant-height high-resolution nc-AFM images of the middle and the zigzag end of a GNR obtained with a CO-terminated tip (AFM set-point offset by 30 pm). (f,g) Constant-height nc-AFM (f) and constant-current STM (g) images of 22 monomer unit long GNR with a single missing benzene ring marked by the red arrow. AFM set-point offset by 48 pm. Inbscale bar, 10 nm, other scale bars, 1 nm. Figure 1: Chemical structure of atomically precise graphene nanoribbons. ( a ) Bottom-up synthesis of an armchair GNR results in zigzag terminated ends. ( b ) STM overview image showing a free GNR ( V =50 mV, I =5 pA). ( c ) Free GNR imaged with a CO-terminated tip ( V =10 mV, I =5 pA). ( d , e ) Constant-height high-resolution nc-AFM images of the middle and the zigzag end of a GNR obtained with a CO-terminated tip (AFM set-point offset by 30 pm). ( f , g ) Constant-height nc-AFM ( f ) and constant-current STM ( g ) images of 22 monomer unit long GNR with a single missing benzene ring marked by the red arrow. AFM set-point offset by 48 pm. In b scale bar, 10 nm, other scale bars, 1 nm. Full size image The electronic structures of defect-free and free-lying GNRs are probed using differential conductance spectroscopy [19] , [20] . In agreement with previous work, we find the onset of the valence and conduction bands at −0.9 and 1.8 V, respectively ( Supplementary Fig. S1 ) [16] . In the following, we focus on the zigzag ends, which are the natural places for contacts. The GNR ends exhibit a localized state with an energy close to the Fermi level [21] . 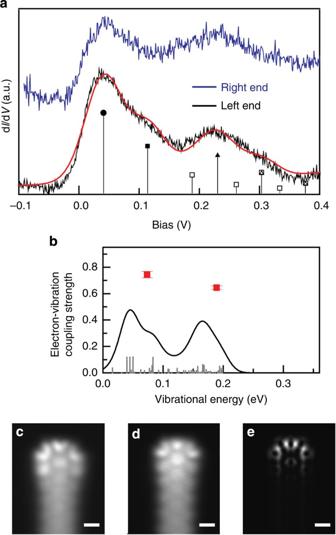Figure 2: Comparison between experimental and calculated vibronic structure. (a) Differential conductance spectra measured on the two ends of an isolated GNR (blue and black lines) fitted with a model for vibronic transport with two vibrational modes with energies of 74 and 189 meV, solid square and triangle, respectively. The elastic peak is indicated by a solid circle. Open symbols correspond to overtones and combination modes. All peaks were broadened by 40 meV and summed up to give the red line. Spectra acquired with a metal tip. (b) Comparison between experimentally determined and calculated e–v coupling strength. The experimental points, as determined from fitting the spectrum inFig. 2a, are indicated by red squares. The calculated e–v coupling constantsλqof all modes (gray lines) were broadened by a gaussian of 15 meV, and summed up (black line). Note that the zero energy corresponds to the energetic position of the elastic peak as determined inFig. 2a. (c,d) Constant-height dI/dVmaps recorded with a CO-terminated tip at the bias voltage corresponding to the elastic peak (c, 50 mV) and to the vibronic replica (d, 225 mV). (e) Corresponding calculated local density of states map assuming that CO-tip can be modelled as a p-wave tip. Scale bars, 0.5 nm. Figure 2a shows d I /d V spectra measured at the two ends of a free ribbon in a small bias range close to the Fermi energy. The resonance at 30 mV has been observed before and is assigned to an end state localized at the zigzag edge [21] . Indeed, this feature is not present in spectra acquired with the tip positioned above the centre of the ribbon ( Supplementary Fig. S1 ). The end state is located at positive bias, implying the GNR to be hole doped by the Au(111) substrate [13] , [16] , [17] , [22] . Its spatial shape can be imaged by taking d I /d V maps in the constant-height mode ( Fig. 2c ). In order to enhance the spatial resolution of the maps, they were obtained with a CO-terminated tip, which gives the tip wavefunction p-wave character [23] . The experimentally observed nodal plane structure is in agreement with the simulated image ( Fig. 2e ). Note that the simulations did not take non-resonant tunnelling into account and used a purely p-wave tip (see Supplementary Note 1 for details) [23] , [24] . Figure 2: Comparison between experimental and calculated vibronic structure. ( a ) Differential conductance spectra measured on the two ends of an isolated GNR (blue and black lines) fitted with a model for vibronic transport with two vibrational modes with energies of 74 and 189 meV, solid square and triangle, respectively. The elastic peak is indicated by a solid circle. Open symbols correspond to overtones and combination modes. All peaks were broadened by 40 meV and summed up to give the red line. Spectra acquired with a metal tip. ( b ) Comparison between experimentally determined and calculated e–v coupling strength. The experimental points, as determined from fitting the spectrum in Fig. 2a , are indicated by red squares. The calculated e–v coupling constants λ q of all modes (gray lines) were broadened by a gaussian of 15 meV, and summed up (black line). Note that the zero energy corresponds to the energetic position of the elastic peak as determined in Fig. 2 a . ( c , d ) Constant-height d I /d V maps recorded with a CO-terminated tip at the bias voltage corresponding to the elastic peak ( c , 50 mV) and to the vibronic replica ( d , 225 mV). ( e ) Corresponding calculated local density of states map assuming that CO-tip can be modelled as a p-wave tip. Scale bars, 0.5 nm. Full size image Electron–vibron coupling Two more peaks are observed in this bias range on the termini of free ribbons. One appears as a shoulder at ~80 mV and the third peak is located at ~220 mV ( Fig. 2a ). The end states of a neutral GNR are predicted to exhibit spin splitting. However, relevant to our experiments, the splitting is predicted to be very small for charged ribbons (calculated levels for neutral and charged ribbons are shown in the Supplementary Fig. S2 ). Therefore, we attribute these peaks to vibronic resonances. Vibronic peaks arise as an electron tunnels through a molecular orbital and simultaneously excites a molecular vibration [25] , [26] , [27] . The energy spacing between the main peak and the first replica corresponds to the energy of that particular molecular vibration. The amplitude of the first replica is directly related to the strength of the e–v coupling [28] , [29] . If the second and third peaks arise from vibronic tunnelling, they should have the same spatial dependence as the elastic resonance. This is confirmed in Fig. 2c , which show d I /d V constant-height maps at voltages corresponding to the first and third peak, respectively. The nodal plane structure observed at 50 and 225 mV is identical. The overall line shape can be fitted well by vibronic transport with two vibrational modes (74 and 189 meV), including overtones and combination modes (red line, Fig. 2a ). The model uses the energies of the modes ħω q and the dimensionless coupling constants λ q as the fitting parameters and the fitted response includes overtones and combination modes as predicted by the theory in Wingreen et al. [28] (see Supplementary Note 2 for details). The results of the fitting procedure with three and four vibrational modes can be found in Supplementary Fig. S3 . The e–v coupling strength can also be calculated theoretically using density functional theory (DFT). The result of such a calculation on a 3 monomer unit long GNR is shown in Fig. 2b . The grey lines indicate the couplings to individual vibrational modes. Broadening the e–v coupling of each mode with a gaussian with a width of 15 meV results in the black line. The overall response has two strong peaks and a shoulder on the lower energy peak. This can be compared with the energies and coupling constants as determined from the experimental d I /d V spectrum. Although the energies are in reasonable agreement, the coupling constants are underestimated by DFT. However, as in reality many modes contribute, the average coupling constant will go down as more modes are included in the fitting of the experimental d I /d V spectrum (see Supplementary Fig. S3 ). One prerequisite to observe vibronic tunnelling is a sufficiently long lifetime of the excited state. In an STM setup, this implies the existence of a double-barrier-tunnelling junction. This is typically realized by inserting a thin layer between the molecule/nanostructure and the metallic substrate [25] , [27] . Here, we observe for the first time vibronic charge transport through a carbon nanostructure adsorbed directly on a metal without the use of spacer groups [30] . This observation supports the notion that the interaction of π-conjugated molecules with Au(111) is weak (no chemical bonding) [18] . Contacting GNRs To study the effect of contacting the GNR to a metal, we controllably created a single GNR-Au bond. An example of such an experiment is shown in Fig. 3 . The middle hydrogen atom at one of the zigzag ends is removed by locally applying a high voltage pulse, similar to the procedures for dehydrogenation of phthalocyanine molecules on Au(111) [31] and benzene on Cu [32] , [33] . 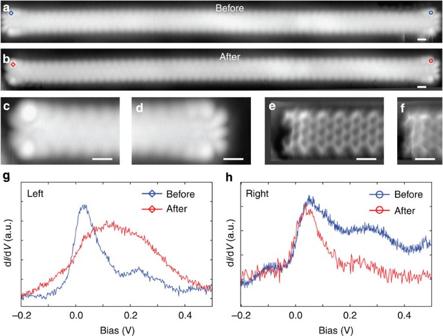Figure 3: Controlled atomic-scale modification of the GNR reduces vibronic coupling. (a) High-resolution STM image of a free GNR (V=50 mV,I=5 pA). (b) High-resolution STM image after a bias pulse has been used to modify the left end of the GNR (V=50 mV,I=20 pA). (c,d) Zoomed-in STM images of the GNR ends after the modification (c:V=50 mV,I=50 pA,d:V=10 mV,I=2 pA). (e) Atomically resolved AFM image of the contacted GNR (AFM set-point offset by 120 pm). (f) AFM image of the same ribbon as ine, but with the tip 80 pm closer to the sample. (g,h) dI/dVspectra recorded at the left and right ends of the GNR before (blue) and after (red) of the modification. All the images and spectra have been acquired with a CO-terminated tip. Scale bar, 0.5 nm. Figure 3a show a free GNR before and after applying a voltage pulse of 3.7 V at the left end of the nanostructure, respectively. After the pulse, the GNRs can no longer be moved laterally, indicating an increased interaction with the substrate. Atomically resolved AFM images show a dark (less repulsive) feature at the position of the middle C atom of the zigzag edge. However, the outer two C 6 rings appear unchanged, that is, similar to the rings in the bulk of the ribbon and to the rings of the intact end. AFM imaging at smaller tip-sample distances reveals bonds in the direction of the middle zigzag C atom ( Fig. 3f ). The above strongly suggests that the middle C atom bent down and formed a bond with the underlying Au(111) substrate. Further evidence on the removal of a single hydrogen atom by voltage pulses comes from experiments on ribbons where the zigzag end does not exhibit the low bias state ( Supplementary Fig. S4 ). Figure 3: Controlled atomic-scale modification of the GNR reduces vibronic coupling. ( a ) High-resolution STM image of a free GNR ( V =50 mV, I =5 pA). ( b ) High-resolution STM image after a bias pulse has been used to modify the left end of the GNR ( V =50 mV, I =20 pA). ( c , d ) Zoomed-in STM images of the GNR ends after the modification ( c : V =50 mV, I =50 pA, d : V =10 mV, I =2 pA). ( e ) Atomically resolved AFM image of the contacted GNR (AFM set-point offset by 120 pm). ( f ) AFM image of the same ribbon as in e , but with the tip 80 pm closer to the sample. ( g , h ) d I /d V spectra recorded at the left and right ends of the GNR before (blue) and after (red) of the modification. All the images and spectra have been acquired with a CO-terminated tip. Scale bar, 0.5 nm. Full size image Higher magnification STM images ( Figure 3c and d ) show how the electronic state on one end is modified by the bonding to the surface, while the spatial shape of the electronic state at the opposite end appears unaltered. Differential conductance spectra taken on the end where the contact was made show only one broad resonance. It is not possible to assess the strength of the vibronic coupling in this ribbon end due to the increased life-time broadening caused by the bond formation. The shift of the peak may be related to p-type doping or to a change in the orbital energy due to the bond formation. Moreover, d I /d V spectra of the opposite (intact) end show that contacting the GNR several tens of nanometres away results in a large decrease in the e–v coupling: the vibronic replicas are strongly suppressed due to formation of a single C–Au bond (at the opposite end). Note that the elastic resonance at the intact end is unchanged. In addition, contacting the GNR does not lead to changes in the conduction and valence bands, demonstrating the electronic structure of the GNR is not affected by contacting ( Supplementary Fig. S5 ). We have created single-atom contacts to four different free ribbons. In all cases, we observed a weakening of the e–v coupling strength. As there is no registry between the ribbons and the Au(111) surface, it is unlikely that the weakening is due to a change of the adsorption site of the GNR. Furthermore, as pointed out above, the ribbons are weakly coupled to the substrate. For such systems, the substrate does not have a large influence on the relative magnitude of the e–v coupling strength (all spectra were acquired at positions with a maximum apparent height [24] ). It is well-known that the lifetime of the electron on a molecular resonance has a significant effect on the vibronic-coupling strength. As the lifetime is shortened, the vibronic features decrease in intensity [29] , in line with our results. In addition, formation of an atomic contact increases dissipation, leading to a faster decay of the vibrationally excited state and to a decrease of inelastic carrier transport [34] . The results shown in Fig. 3 demonstrate that the strength of the e–v coupling and the electron lifetime are sensitive to the exact atomic-scale structure of the GNRs. To investigate these effects in more detail, we examine a GNR that is most likely connected in the middle to another ribbon ( Fig. 4a ). In turn, this second ribbon is part of a large network of connected species. Such structures occur naturally after the on-surface polymerization and cyclodehydrogenation steps. Although the elastic peak position and amplitude and wavefunction structure at the ends of the ribbon are very similar to an isolated GNR, the vibronic peaks are very weak (see Fig. 4c ). This suppression of the e–v coupling is likely to be caused by a similar mechanism as in the case of contacting individual ribbons: the lifetime of the vibrationally excited state is reduced either owing to increased tunnelling rate out of the GNR or increased energy dissipation owing to better coupling with the phonons of the substrate or the neighbouring ribbon. 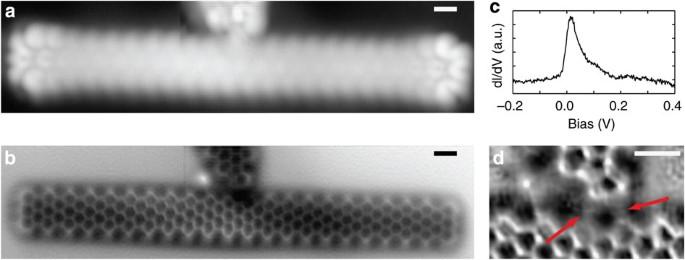Figure 4: Chemical and electronic structures of commonly observed defects. (a,b) STM (a) and AFM (b) images recorded with a CO-terminated tip of a GNR connected in the middle by another ribbon (STM setpoint:V=10 mV,I=15 pA. AFM offset w.r.t. STM: 30 pm). (c) dI/dVspectra acquired on the end of the ribbon shown ina(with a CO-tip). (d) Higher magnification constant-height AFM image of the junction shown in (b) (local contrast). AFM set-point offset by 50 pm. Arrows indicate possible bonds between the ribbons. In all cases, scale bar, 0.5 nm. Figure 4: Chemical and electronic structures of commonly observed defects. ( a , b ) STM ( a ) and AFM ( b ) images recorded with a CO-terminated tip of a GNR connected in the middle by another ribbon (STM setpoint: V =10 mV, I =15 pA. AFM offset w.r.t. STM: 30 pm). ( c ) d I /d V spectra acquired on the end of the ribbon shown in a (with a CO-tip). ( d ) Higher magnification constant-height AFM image of the junction shown in ( b ) (local contrast). AFM set-point offset by 50 pm. Arrows indicate possible bonds between the ribbons. In all cases, scale bar, 0.5 nm. Full size image We have demonstrated that defect-free GNRs show a mid-gap state localized on the zigzag termini, as well as valence and conductions states in agreement with DFT. The GNRs are weakly coupled to the Au(111) substrate. Au–C bonds can be created at well-defined positions by removal of a single hydrogen atom through a voltage pulse from the STM tip. By directly comparing the electronic structure of a ‘free’ GNR with the electronic structure of the same ribbon after making contact with the metal substrate, we obtain direct and unambiguous information on the effect of coupling to the leads. This approach should be generally applicable to study the effect of contact formation. We find that creating a single carbon-metal bond does not modify the bulk electronic structure (valence and conduction bands) of the GNR, but strongly reduces the strength of the electron–vibration coupling of the end state due to an increased coupling with the substrate. This effect can be sensitively probed by measuring the amplitude of the vibronic replica, that is, the intensities of inelastic transport signatures. Sample preparation The 10-10′-dibromo-9-9′ bianthryl molecules were synthesized by subsequent decomposition of the Grignard of 9-bromo-anthracene over CuCl 2 followed by bromination using bromine [13] , [35] . Samples were prepared by evaporating the bianthryl precursor molecule from a Knudsen cell-type evaporator onto a Au(111) single crystal cleaned by standard procedures and two subsequent heating steps [13] , [17] . This resulted in a sub-monolayer coverage with a low number of free GNRs. STM and AFM measurements After the growth, the sample was inserted into a low-temperature STM/AFM ( T =4.8 K, Omicron LT-STM/QPlus AFM), housed within the same ultrahigh vacuum system (base pressure <10 −10 mbar). We used a QPlus sensor with a resonance frequency f 0 of 24,454 Hz, a quality factor of 12,227, and a peak-to-peak oscillation amplitude of ~86 pm. STS measurements were performed using a lock-in amplifier (frequency=714 Hz, amplitude=10 mV (rms)). Picking up an individual carbon monoxide molecule to the tip apex was used to achieve atomically resolved AFM images and to improve the spatial resolution of STM orbital imaging [23] , [36] , [37] . For the constant-height AFM images, the tip-sample distance was typically decreased by a few tens of pm (as indicated in the figure captions) w.r.t. the STM set-point ( V =50 mV, I =10 pA) after switching off the feedback. AFM images were recorded with V =0 V. How to cite this article : van der Lit, J. et al. Suppression of electron–vibron coupling in graphene nanoribbons contacted via a single atom. Nat. Commun. 4:2023 doi: 10.1038/ncomms3023 (2013).